In situelectron holography study of charge distribution in high-κcharge-trapping memory Charge-trapping memory with high- κ insulator films is a candidate for future memory devices. Many efforts with different indirect methods have been made to confirm the trapping position of the charges, but the reported results in the literatures are contrary, from the bottom to the top of the trapping layers. Here we characterize the local charge distribution in the high- κ dielectric stacks under different bias with in situ electron holography. The retrieved phase change induced by external bias strength is visualized with high spatial resolution and the negative charges aggregated on the interface between Al 2 O 3 block layer and HfO 2 trapping layer are confirmed. Moreover, the positive charges are discovered near the interface between HfO 2 and SiO 2 films, which may have an impact on the performance of the charge-trapping memory but were neglected in previous models and theory. Charge-trapping memory (CTM) with high- κ dielectric substituting floating gate as the charge capture layer is a candidate for next-generation storage devices as it radically improves the retention force, weakens the coupling effect and the charge leakage. The elusive spatial charge distribution in the CTM has an important role influencing the programme/erase speed and the retention force. Therefore, it is critical to map the charge distribution in the dielectric layers to clear the trapping mechanism of CTM and improve the design and fabrication process to ensure the performance of the future memory devices. I–V and C–V measurements are the usual characterization tools to deduce the charge distribution along vertical direction of the charges with the appropriate models. However, these methods concerning models only depict the effective charge distribution with a poor spatial resolution and moreover, these indirect electrical investigations can be disturbed so easily by the measurement environment or parameters that controversial results were reported in the literatures. You et al . [1] thought that the electrons were bulk trapped in the HfO 2 trap layer but interface trapped in the Si 3 N 4 trap layer. Zhu et al . [2] indicated that the trapped charges located in both interface and bulk in the HfO 2 layer. Bu and White [3] found that the charges concentrated on the interface between the block and trap layer, whereas Zahid et al . [4] reported that electrons aggregated in the interface between the metal gate and block Al 2 O 3 layer and those electrons could vary the threshold voltage, which was confirmed by Rao et al . [5] and Padovani et al . [6] Sharma et al . [7] showed that the holes generated in the SiO x N y trap layer might cause the profiled electron centroid moving towards the HfO 2 block layer. Ko et al . [8] pointed that oxygen interstitials or Hf vacancies, beside the oxygen vacancies, may have the important roles as the charged point defects in charge-trapping process. Ramanathan et al . [9] noted that the C–V curve could not perfectly reflect the charge-trapping phenomena because of the complexity of test environment. Recently, several types of scanning probe microscopy (SPM), such as electrostatic force microscope [10] , Kelvin force microscope [11] , scanning capacitance microscope [12] and conductive atomic force microscope [13] , have been used to profile the charge distribution in CTM with tens of nanometre resolution. SPM can track the lateral charge map and diffusion process but the working mode and the limited spatial resolution impede it to distinguish the vertical location of the trapped charges, which have an impact significantly on the performance of the device. Therefore, a direct observation is urgently needed to clarify the charge location in CTM. Electron holography is a powerful means to image the electrostatic potential distribution because the charges in the sample can alter the phase of the penetrated electron wave and such phase disturbance can be retrieved from the electron interference patterns. Electron holography in transmission electron microscope (TEM) has been employed to map the depletion layer in p – n junction [14] , the interfacial polarization field in the superlattices [15] , two-dimensional electron gas and two-dimensional hole gas in the high electron mobility transistor device [16] and the charge distribution in nanomaterials [17] . Combined with in situ techniques, the bias-induced potential variations in p – n junction [18] and metal oxide semiconductor (MOS) transistor [19] were imaged. It should be noted that electron holography in TEM possesses the merit to snapshot the potential image with high spatial resolution, which is extremely important for the characterization of nanometre materials and devices. In this paper, in situ electron holography in TEM has been adapted to map the vertical and lateral charge distribution within the CTM simultaneously. Benefited by the high-resolution electron holography, the charge-trapping process traced under different gate biases indicates unambiguously that the electrons penetrate through the HfO 2 layer and aggregate beneath the interface between HfO 2 and Al2O 3 films. Structure and in situ I–V characterization The schematic diagrams of the in situ measurements and the hologram acquirements are shown in Fig. 1a,b , respectively. Conventionally, the reference wave in electron holography is the beam passing through the vacuum. However, in principle every wave with known or invariant phase distribution, for example, the electron beam penetrating the Al gate layer here, is also available to preserve the relative phase difference feature between the insulator layers and the Si substrate [20] , [21] , as discussed in Method. A low-magnification cross-section image ( Fig. 2a ) depicts the multilayer stacks of the CTM sample fabricated by focused ion beam (FIB) technology (see Supplementary Fig. S1 ) and the high-magnification image ( Fig. 2c ) show the abrupt interfaces between the functional films where the HfO 2 layer is polycrystalline (P2 1 /c, a =5.117 Å, b =5.175 Å, c =5.291 Å, α =90°, β =99.216°, γ =90°; polycrystalline morphology is shown in Supplementary Fig. S2 ). Those HfO 2 grains with different orientation may induce various dynamic diffraction phase as the uneven feature in the phase map of the HfO 2 layer without bias ( Fig. 2d ). The I–V curve of the pristine sample in the wafer test ( Fig. 2b ) indicates that current tunnelling or electron injecting erupts above 5 V, whereas the C–V measurement shows a discernible storage winder opened at 8 V (see Supplementary Fig. S3 ). Considering the background current of the galvanometer, in situ electric measurements of the FIB-cutting sample in TEM from a wafer different to ‘wafer test’ one, with and without electron beam illuminating, demonstrate the similar charging behaviour and apparently the electron beam shower has the negligible impact on in situ test results. 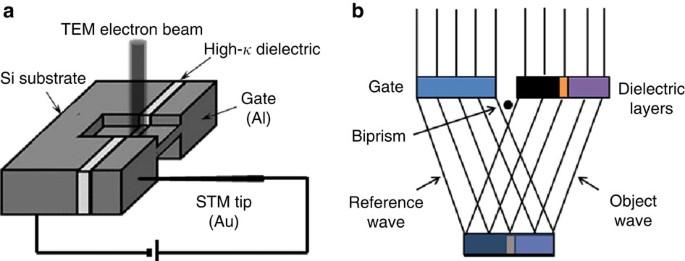Figure 1: Schematic diagrams ofin situTEM electron holography. (a) The set-up of thein situexperiment, (b) the optical principle of electron holography. Figure 1: Schematic diagrams of in situ TEM electron holography. ( a ) The set-up of the in situ experiment, ( b ) the optical principle of electron holography. 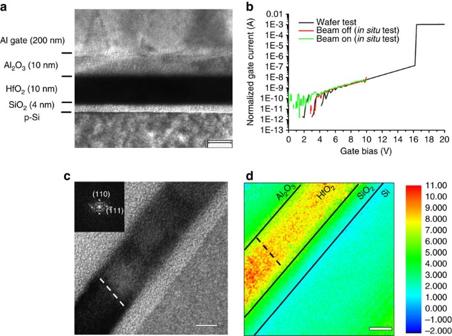Figure 2: Structure and I–V behaviour of the CTM sample. (a) The low-magnification cross-section image of the CTM sample. (b) The normalized I–V curves measured on the wafer and in TEM, with and without electron beam illumination (black: wafer test, red:in situtest with beam off, green:in situtest with beam on). (c) The high-magnification image of the polycrystalline HfO2layer, the insert is the fast Fourier transform of one HfO2grain. (d) The phase image of the unbiased CTM sample involving the three dielectric stacks and the Si substrate; the uneven phase in HfO2layer come from the polycrystalline feature. The dashed lines incanddindicate the position of grain boundary. Scale bar, 10 nm (a), 5 nm (b), 5 nm (c). Full size image Figure 2: Structure and I–V behaviour of the CTM sample. ( a ) The low-magnification cross-section image of the CTM sample. ( b ) The normalized I–V curves measured on the wafer and in TEM, with and without electron beam illumination (black: wafer test, red: in situ test with beam off, green: in situ test with beam on). ( c ) The high-magnification image of the polycrystalline HfO 2 layer, the insert is the fast Fourier transform of one HfO 2 grain. ( d ) The phase image of the unbiased CTM sample involving the three dielectric stacks and the Si substrate; the uneven phase in HfO 2 layer come from the polycrystalline feature. The dashed lines in c and d indicate the position of grain boundary. Scale bar, 10 nm ( a ), 5 nm ( b ), 5 nm ( c ). Full size image Characterizing the charge location After stripping off the inner potential and the dynamic diffraction effect, bias-induced phase features Δ φ bias ( x , y ) of the high- κ dielectric HfO 2 layer together with the whole SiO 2 interlayer, parts of Al 2 O 3 block layer and Si substrate readily display the phase evolution in the HfO 2 layer under different bias ( Fig. 3 ). The projected charge density maps calculated from the second differential of Δ φ bias ( x , y ) images are shown in Fig. 4 , with the relative permittivities of 9 for Al 2 O 3 , 20 for HfO 2 , 3.9 for SiO 2 and 11.7 for Si. The projected charge density maps illustrate unambiguously that the charges aggregate unevenly and diffuse laterally within the HfO 2 layer with increasing bias. The negative charge centroid locates near the interface between the HfO 2 film and the Al 2 O 3 and lateral migration is also along this interface where a large amount of traps may exist there. 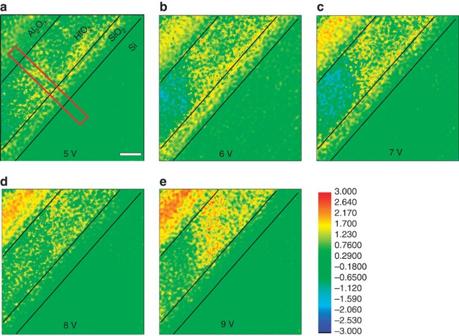Figure 3: Bias-induced phase feature Δφbias(x,y) under different bias. (a) 5 V, (b) 6 V, (c) 7 V, (d) 8 V, (d) 9 V. Scale bar, 5 nm. Figure 3: Bias-induced phase feature Δ φ bias ( x , y ) under different bias. ( a ) 5 V, ( b ) 6 V, ( c ) 7 V, ( d ) 8 V, ( d ) 9 V. Scale bar, 5 nm. 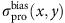Figure 4: Projected charge densitymaps under different bias. (a) 5 V, (b) 6 V, (c) 7 V, (d) 8 V, (d) 9 V. The top-left Al2O3layer locates in the Fresnel stripes of the hologram; hence, its second differential result may deviate from the true value in some degree. The inversed layer ofp-Si can be observed beneath the SiO2film as a slight negative stripe. The dashed lines indicate the position of grain boundary, as shown inFig. 2c,d. Scale bar, 5 nm. Full size image Figure 4: Projected charge density maps under different bias. ( a ) 5 V, ( b ) 6 V, ( c ) 7 V, ( d ) 8 V, ( d ) 9 V. The top-left Al 2 O 3 layer locates in the Fresnel stripes of the hologram; hence, its second differential result may deviate from the true value in some degree. The inversed layer of p -Si can be observed beneath the SiO 2 film as a slight negative stripe. The dashed lines indicate the position of grain boundary, as shown in Fig. 2c,d . Scale bar, 5 nm. Full size image An interesting feature is the positive charges locating near the interface between HfO 2 and SiO 2 films. Usually, the external voltage applied to the dielectric capacitor could cause the negative/positive dipole layer whose positive charges locate near the cathode, whereas the negative charges place beneath the anode, which is out of the observation field. In addition, tunnelling current inducing positive charges (or current-generated positive charges), which have been studied abundantly in the SiO 2 gate insulator of the MOS structures since the early 1980s should be another important source [22] , [23] . It is speculated indirectly from the electric measurements that the positive charges can be generated and even become the overwhelming trapped charges in the SiO 2 film when tunnelling electrons pass through the gate insulator [22] , [23] . Similar behaviour was also observed in high- κ stack MOS devices [7] , [24] , [25] . To rule out the parasitic dipoles and grasp a semiquantitative estimation of the injected charge distribution, the line phase profiles averaged in the rectangle of each phase map have been fitted with COMSOL Multiphysics simulation software under Gaussian distribution assumption of the injected electrons and current-generated positive charges (see Methods). The fitted curves ( Fig. 5 ) coinciding well with the experimental data supply the quantitative estimation of the charge distribution and the variation with bias change. The charge distribution excluding the dipolar charges as well as the net charges and the effective charge density from the fitted data are plotted in Fig. 6 . Although the centroid of the projected charge density in Fig. 4 seems on the top of the HfO 2 film, the simulated results display thoroughly that the centroid should be near the interface between Al 2 O 3 block layer and HfO 2 trapping layer. The possibility of negative charge trapping in the middle of HfO 2 or in the interface between HfO 2 and SiO 2 could be excluded here. As expected, the effective charges are negative although the mount of positive charges grows simultaneously. It also explains why those positive charges are seldom recognized in the charge-trapping process characterized with traditional electric measurement, which can only detect the effective or net charges and conceal the existence of positive charges. Now, not only the exact location of the negative charges but also the figure of the positive charges is visualized in the dielectric stacks with high spatial resolution. The inversed layer generated within the p -Si substrate also appears as a slight negative stripe beneath the SiO 2 dielectric film. The results also demonstrate that electron holography can detect several hundreds of electrons within a small region. 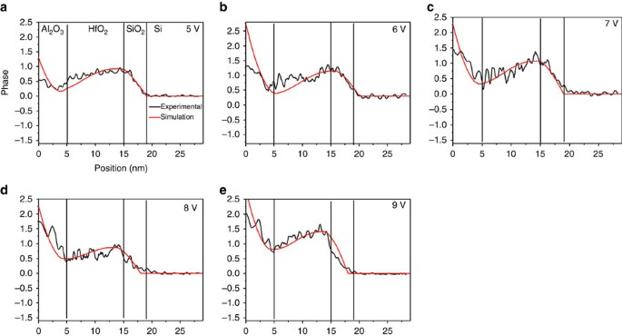Figure 5: Experimental and the simulated phase profiles. (a) 5 V, (b) 6 V, (c) 7 V, (d) 8 V, (e) 9 V. Experimental data are averaged from the rectangles inFig. 3, plotted with simulated phase curve. The flat phase in the Si region confirms the uniform thickness of the sample. Figure 5: Experimental and the simulated phase profiles. ( a ) 5 V, ( b ) 6 V, ( c ) 7 V, ( d ) 8 V, ( e ) 9 V. Experimental data are averaged from the rectangles in Fig. 3 , plotted with simulated phase curve. The flat phase in the Si region confirms the uniform thickness of the sample. 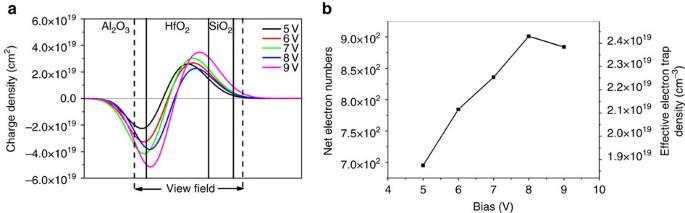Figure 6: Negative and positive charge distribution. (a) Charge distribution for the simulation and (b) corresponding net charges and effective charge density in the whole stacks. Full size image Figure 6: Negative and positive charge distribution. ( a ) Charge distribution for the simulation and ( b ) corresponding net charges and effective charge density in the whole stacks. Full size image Charging process Subsequently, the charging scenario can be portrayed based on the above results. Under a lower bias, the Fowler–Nordheim tunnelling mechanism occurs, although the situation is more complicated in HfO 2 stacks than in pure SiO 2 film [26] . The band diagram is shown in Supplementary Fig. S4 . The tunnelling electrons move towards the anode and the positive charges generated by trap creation, impact ionization [27] , or the defects in the HfO 2 layer [28] , [29] , [30] , [31] , [32] move oppositely. The hydrogenous species releasing hydrogen in the insulator HfO 2 or SiO 2 may be another source of the positive charges [33] . The possibility of gate-injected holes could be ruled out as the distance between the gate and Si substrate is 24 nm and the injected holes may be neutralized halfway and cannot aggregate on the observed place. Different from the thin-SiO 2 -film MOS transistor where the tunnelling electrons are absorbed immediately by the anode gate, part of the tunnelling electrons would be blocked beneath the Al 2 O 3 layer, whereas the positive charges would be trapped a tunnelling distance above the Si surface [27] . Some positive charges will tunnel back to the substrate under the positive gate bias. The reported 5 nm tunnelling distance of those positive charges under low bias press [34] indicates that the residual positive charges should be 5 nm above the silicon substrate, or just 1 nm above the 4 nm SiO 2 interlayer, consistent with the observed positive charge location. With increasing bias, an amount of tunnelling electrons may pour into the HfO 2 layer through some weak points in the SiO 2 film. The degradation spots in the thin SiO 2 film due to local soft breakdown [27] or progressive breakdown [35] by positive charge may be another possible injection point. The electrons would migrate vertically faster along the HfO 2 grain boundary [36] , [37] , [38] because of the higher vertical electric strength so that the electrons aggregate first beneath the Al 2 O 3 block layer and later diffuse along the interface between Al 2 O 3 and HfO 2 , as demonstrated sequentially in Fig. 4 . The positive charges trapped near the bottom of HfO 2 cannot be neutralized completely at once, as both injection channel and electron diffusion are spatially limited and inhomogeneous, although the total negative charges surpassing the positive charges result in the net electrons trapping throughout the C–V or I–V characterization. The coexistence of the negative and positive charges cannot be discerned by general electric diagnoses, which feature the effective charge behaviour only as well as SPM with charge force detector whose resolution is too poor to distinguish the vertical charge spatial separation. The positive charge layer neglected in the previous pr ogramming studies with or without modelling analysis should be taken seriously because it may have a contradictory role that not only enhances the electron tunnelling through SiO 2 film to accelerate the charging process [26] but also increases the risk of SiO 2 breakdown and the retention charge loss [39] , affecting the programming/erasing performance and the device reliability [40] , [41] . The uneven distribution of the positive and negative charges may reflect that the charge traps do not distribute uniformly in the nanoscale because of the grains in the HfO 2 layer, although the local morphology of the interface seems flate. Influence of illuminating electron beam The high-energy (200 kV) electrons of the illuminating beam could be trapped or produce holes in the dielectric layers, which may be involved in the charge distribution. However, the number of those electrons or holes should be invariable because of the fixed dose of illumination; hence, it is hard to attribute the change of the charges’ amount and location in Figs 3 and 4 to the impact of the high-energy electron beam. The charges’ evolution and their location in the sample studied here may be also influenced by the surface depletion in the thin TEM sample as well as the unavoidable FIB-cutting damage, which possibly induces SiO 2 degradation or causes the larger current leakage, deviating from the pristine materials. Considering the physical or chemical sculpturing process during devices fabrication and the tiny size of the next-generation memory unit, the charge-trapping behaviour revealed with the in situ electron holography here still shows the significance to the future actual memory devices. The phase images acquired under different illumination dose also confirm that the intensity of the electron shinning beam can be neglected compared with the bias effect (see Supplementary Fig. S5 ). Recombination without bias Another noteworthy point is that the bias is no more than 9 V in this paper because of the voltage ceiling of the in situ voltmeter. If the bias press increases higher, the injected electrons should fill more part of the interface between HfO 2 and SiO 2 . However, whether the positive charges are annihilated completely is yet to be confirmed in future. Further, not the charge retention location but the charging process is monitored here. If the bias disappears, the negative and positive charges could recombine to result in a redistribution of charges [42] , and it may be in a steady-state manner different from the observation here. Charge-pumping method [43] is more sensitive to the surface state, so it is employed to find the charges trapped on or close to the interface between SiO 2 and the trap layer [44] , [45] , but it is difficult to detect the negative charges locating deeply in the HfO 2 layer. Transient analysis method can demonstrate the centroid of the charges not only on the interfaces but also inside the trap layer [46] , [47] . However, it could not display the spatial details about the charges’ distribution and relationship between such distribution and the device morphology. Here in situ electron holography visualizes the detailed scenery of the local charge distribution and its evolution in the high- κ charge-trapping devices under varied bias for the first time. The extracted phase changes induced by bias stress with high spatial resolution reveal the coexistence of the negative and positive charges during charging process, which was neglected by the previous electric characterization and theory analysis. The electrons injected under higher bias may pass through the HfO 2 grain boundary and accumulate near the interface between Al 2 O 3 and HfO 2 dielectric layers, whereas the positive charges are trapped in the interface between the HfO 2 and SiO 2 films. The discovered positive charges that have been studied in the SiO 2 gate insulator for many years are seldom considered in electron tunnelling of high- κ CTM structures before but should arise enough attention as the positive charges may influence the device performance, especially the lifetime as well as the impact on the breakdown of the anodic SiO 2 in MOS structures. The species of the positive charges and the relationship between the inhomogeneous electron injection and the uneven structure features of HfO 2 film should be clarified by the on-going work. The trapping level of the charges revealed that the in situ electron holography should also be analysed combined with other methods, including theory calculation, in future works. The studied HfO 2 trapping structures are something different with the silicon–oxide–nitride–oxide–silicon systems; thus, the charge distribution uncovered here may be not as same as in the silicon–oxide–nitride–oxide–silicon devices. High- κ charge memory sample The HfO 2 -based CTM sample was prepared as follows. The p -type Si (100) wafers with a resistivity of 8–12 Ω were cleaned by the standard Radio Corporation of America process. Then, a 4-nm SiO 2 film acting as the tunnelling layer was thermally grown in dry O 2 ambience. Two layers of Al 2 O 3 and HfO 2 with thicknesses of 10 nm were deposited sequentially on the SiO 2 film. All the films were deposited in situ by atomic layer deposition at a substrate temperature of 250 °C. Post-deposition annealing process was carried out in N 2 ambience under 700 °C for 1 min. Finally, a 200-nm thick Al gate electrode was formed by a lift-off process. In situ holography characterization The CTM samples were mechanically milled and then cut by FIB with ±2° refinement to guarantee the uniform thickness. Additional 5 s ion milling was performed to remove the surface amorphous layers and the possible dead layers. The thickness of the sample for holography study was about 150 nm, characterized with electron energy loss spectroscopy (see Supplementary Fig. S6 ), which agrees well with the measurement in SEM image (see Supplementary Fig. S1c ). The sample was installed on a Nanofactory in situ holder, which can manipulate the Au tip to apply the voltage to the Al gate of the sample and monitor the current at the same time. Electron holograms were recorded in charge-coupled device camera of Tecnai F20 electron microscope equipped with holography biprism. Standard vacuum reference hologram was pictured first to correct the phase distortion from the optical system while the in situ electron holograms were recorded with the reference wave penetrating the Al gate because the limited view field of hologram at high magnification cannot place the vacuum region over the interesting high-κ layers buried deeply below the Al gate. The reference hologram ( Supplementary Fig. S7a ) is used to estimate the spatial resolution. The sideband location in the fast Fourier transform of the reference hologram ( Supplementary Fig. S7b ) corresponds to a 0.22-nm resolution ( ). Not in the most cases but is employed to reconstruct the phase image to improve the signal-to-noise ratio, and thus the retrieved spatial resolution is down to about 1 nm, which is enough for the investigation. The holography reconstruction is completed with the plug-in HoloWork in Digital Micrography of Gatan, and the unwrapping processing is achieved with a published code [48] . The contrast of the interference fringes in the sample hologram is also degraded from 8 to 3.5% because of the deterioration of the beam coherence. Therefore, many extracted phase images are averaged to obtain the enough phase resolution ( Supplementary Fig. S7c,d ). For a sample, the image processing to extract the bias-induced phase map Δ φ 5 V ( x , y ) is shown here. Δ φ 5 V ( x , y ) ( Fig. 3a ) is calculated by Supplementary Fig. S8 subtracting Supplementary Fig. 2d directly after the image alignment. As discussed below, using electron beam from Al gate as reference wave will not confuse the analysis of charge-induced phase modulation in the high- κ dielectric film. It also avoids the risk of stray field disturbance in the conventional scheme where the phase of the vacuum reference wave could be distorted by the stray field of gate or electrode [49] but the phase resolution is sacrificed because of the coherence deterioration of the penetrating wave [50] . Thus, at least 20 retrieved phase images for each bias were averaged to obtain the final phase distribution, including 0 V image, which was subtracted as the ‘background’ from the phase maps under bias. The statistical s.d. 0.1 in the Si substrate in Fig. 3a could be an estimation of the phase resolution here because the bias-induced phase in the grounded Si substrate should be a constant. The sample drift was corrected by post-alignment of holograms with the mark in the sample. Thus, the resulted image size was only 805 × 823 pixels although the original image size was 1,024 × 1,024 pixels. The gate bias was kept during the acquirement of the hologram. The phase distribution of the reconstructed image including the dielectric stacks and Si substrate without gate bias φ 0 V ( x , y ) is determined by the phase difference between the objective phase containing and and the reference gate phase involving and , where ‘iner’ and ‘dyn’ indicate the mean inner potential and the possible dynamic diffraction effect, respectively. It is apparent that , , and are the intrinsic physical property of the sample and the orientation correlated effect, which do not vary under bias. When a bias is applied to the gate, the phase φ bias ( x , y ) should be changed to where is the phase shift caused by the trapped charges and is the additional phase by the bias. Thus, the reconstructed contains not only the features induced by the gate bias but also the contributions of the mean inner potential and the dynamic diffraction similar to φ 0 V ( x , y ). After a careful image alignment, φ 0 V ( x , y ) could be subtracted from and then the bias-induced phase feature Δ φ bias ( x , y ) should be, It is reasonable to assume that the bias-caused phase shift should be a constant or acts as a uniform phase background because the metal gate could be regarded as an equipotential under given bias. Therefore, Δ φ bias ( x , y ) could be presented as where is substituted by and , indicating the phase shift of Si substrate and the dielectric layers in the view field, respectively. The attention is focused on the phase shift of the insulator stacks because may also be an invariant feature because of the grounded Si substrate, confirmed by the flat phase configuration of Si in Figs 3 and 5 . Further, the expression of Δ φ bias ( x , y ) is very simple now: where C E is 0.0073/(V nm) for 200 kV electrons, is the ‘projected’ (along electron beam direction z ) potential induced by bias in dielectric layers and t is the sample thickness measured with EELS, 150 nm. Thus, the charge distribution would also result in a strong phase change predominantly in the insulator films, as shown in Fig. 3 . According to the Poisson equation, the projected charge density in the dielectric layer is [51] where ε is the dielectric constant. Therefore, the lateral- and vertical-projected charge density distribution could be extracted directly from the second differential of Δ φ bias ( x , y ) map. Simulation The multilayer model for simulation is shown in Supplementary Fig. S9 . The Gaussian distribution is assumed both for negative and positive charges in the HfO 2 layer. The relative permittivities are 9 for Al 2 O 3 , 20 for HfO 2 , 3.9 for SiO 2 and 11.7 for Si. For the lack of the information from the negative charges due to the polarization, the invariable negative charge density 5 × 10 19 cm −3 has been assumed in the Al 2 O 3 block layer for the convenience. How to cite this article: Yao, Y. et al . In situ electron holography study of charge distribution in high- κ charge trap memory. Nat. Commun. 4:2764 doi: 10.1038/ncomms3764 (2013).